Persistent 400,000-year variability of Antarctic ice volume and the carbon cycle is revealed throughout the Plio-Pleistocene Marine sediment records from the Oligocene and Miocene reveal clear 400,000-year climate cycles related to variations in orbital eccentricity. These cycles are also observed in the Plio-Pleistocene records of the global carbon cycle. However, they are absent from the Late Pleistocene ice-age record over the past 1.5 million years. Here we present a simulation of global ice volume over the past 5 million years with a coupled system of four three-dimensional ice-sheet models. Our simulation shows that the 400,000-year long eccentricity cycles of Antarctica vary coherently with δ 13 C data during the Pleistocene, suggesting that they drove the long-term carbon cycle changes throughout the past 35 million years. The 400,000-year response of Antarctica was eventually suppressed by the dominant 100,000-year glacial cycles of the large ice sheets in the Northern Hemisphere. There have been numerous efforts to explain climate variability during the Cenozoic era, the past 65 million years (Myr). The interactions between orbital forcing, temperature, the carbon cycle and glaciation at high latitudes seem to play important roles in determining the pacing of ice sheets, the variability of the surface-air temperature over the Earth and atmospheric CO 2 concentrations (pCO 2 ) [1] , [2] . For the past ~1 Myr, observations of pCO 2 have shown that temperature and pCO 2 vary coherently over glacial cycles [3] . However, the precise contribution of different components of the climate system to glacial–interglacial variability has yet to be resolved [4] . Although a clear link between changes in solar insolation and ice volume has been determined [5] , [6] , the exact causes and links with the pacing of the carbon cycle and the role of the ocean [7] are not yet fully understood. Ice sheets have been a significant part of the climate system since the transition from the Eocene to the Oligocene (~34 Myr ago). This transition has been identified in the marine sediment records of benthic oxygen isotopes (δ 18 O) as the initiation of Antarctic glaciation [8] , triggered by a decrease in pCO 2 (ref. 9 ). During the Oligocene to Middle Miocene time interval, eccentricity cycles of 100,000-yr (100-kyr) and 400-kyr have been found in multiple marine sediment isotope records of carbon (δ 13 C) and oxygen (δ 18 O) isotopes and have been linked to changes in ice volume and the carbon cycle [1] , [10] , [11] , [12] . Over the past 5 Myr, oceanic carbon isotope records also reveal 400-kyr eccentricity cycles in the global carbon reservoir [13] . In contrast, the absence of the 400-kyr-long eccentricity signal in the Pleistocene ice-age records such as benthic δ 18 O data has raised the so-called ‘400-kyr problem’ [14] . The benthic δ 18 O data are crucial in the interpretation of the long-term environmental changes as it reflects variations in global ice volume and deep-water temperature [15] . Here we use a stacked record of benthic δ 18 O data [16] (LR04) that represents a global averaged signal of climate variability for the Plio-Pleistocene ( Fig. 1a ). We use an inverse forward modelling approach to derive ice volume and temperature from the benthic δ 18 O data over the past 5 Myr. A Northern Hemisphere (NH) temperature anomaly is derived from the difference between modelled and observed benthic δ 18 O data (see Methods). This temperature anomaly is forwarded to four sophisticated three-dimensional (3D) ice-sheet-shelf models and a deep-water temperature parameterization [17] to determine the temperature and ice-volume contributions to the benthic δ 18 O data. The modelled benthic δ 18 O data are calculated by minimizing the difference between the modelled and observed δ 18 O. The coupled system includes four ice-sheet-shelf models that simulate glaciation on Eurasia, North America, Greenland and Antarctica, thereby explicitly calculating all ice-volume contributions separately for the first time over the past 5 Myr. To investigate the disappearance of the 400-kyr-long eccentricity cycles in the benthic δ 18 O data, we analyse the ice-volume simulations and compare these with available proxy data. We show that the 400-kyr-long eccentricity cycles found in Antarctic ice volume, as a result of insolation-driven sub-shelf melting, can be linked to changes in the carbon cycle (δ 13 C) during the Plio-Pleistocene. The emergence of the large NH ice sheets, which are surface mass balance (SMB)-driven, suppresses the 400-kyr-long eccentricity signal in the benthic δ 18 O data. 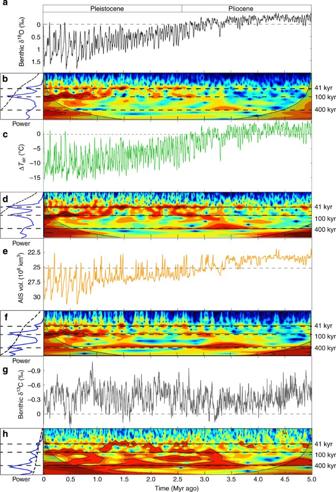Figure 1: Simulated variables and proxies with frequency wavelets. (a) Forcing record of the inverse routine, the LR04 benthic δ18O stacked record16. (b) Wavelet analysis48of LR04. (c) Simulated surface-air temperature anomaly (°C) over Antarctica and (d) wavelet analysis of temperature. (e) Simulated Antarctic ice volume (106km3) and (f) wavelet analysis of ice volume. (g) Eastern equatorial Pacific Leg 138 benthic δ13C record13and (h) wavelet analysis of δ13C. Forb,d,f,h, the >95% confidence levels are indicated by the black lines, and horizontal dashed lines indicate the 41, 100 and 400 kyr frequencies. The light shading indicates possible distorted results due to edge effects of the time series. On the left, the total power spectrum with the 95% confidence level indicated by the dashed line. Figure 1: Simulated variables and proxies with frequency wavelets. ( a ) Forcing record of the inverse routine, the LR04 benthic δ 18 O stacked record [16] . ( b ) Wavelet analysis [48] of LR04. ( c ) Simulated surface-air temperature anomaly (°C) over Antarctica and ( d ) wavelet analysis of temperature. ( e ) Simulated Antarctic ice volume (10 6 km 3 ) and ( f ) wavelet analysis of ice volume. ( g ) Eastern equatorial Pacific Leg 138 benthic δ 13 C record [13] and ( h ) wavelet analysis of δ 13 C. For b , d , f , h , the >95% confidence levels are indicated by the black lines, and horizontal dashed lines indicate the 41, 100 and 400 kyr frequencies. The light shading indicates possible distorted results due to edge effects of the time series. On the left, the total power spectrum with the 95% confidence level indicated by the dashed line. Full size image Simulated climate variability over the past 5 Myr As expected, the LR04 benthic δ 18 O stack [16] shows a strong periodicity in the 41-kyr obliquity band and 100-kyr glacial periodicity during the past 1 Myr ( Fig. 1a,b ). The 400-kyr-long eccentricity cycles in benthic δ 18 O data are much less pronounced throughout the past 5 Myr ( Fig. 1b ). Reconstructed temperature ( Fig. 1c,d ) exhibits a similar periodic behaviour as the benthic δ 18 O data ( Supplementary Fig. S1 and Supplementary Data 1 ). However, simulated Antarctic ice volume ( Fig. 1e,f ) does reveal a significant and persistent 400-kyr periodicity, responding to long eccentricity variability in the sub-ocean shelf melt ( Supplementary Fig. S2b,d ). In particular, the 400-kyr periodicity is found in ice discharge ( Supplementary Fig. S2f ). For the Antarctic ice sheet (AIS), it is the dominant frequency for the period from 4.2 to 3 Myr before present ( Fig. 2b ). 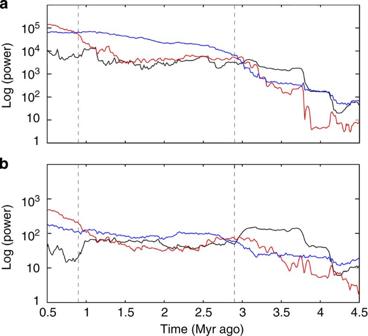Figure 2: Power evolution in eccentricity and obliquity frequency bands. For both panels, 400-kyr power is shown in black, 100-kyr power in red and 41-kyr power in blue. (a) Eustatic sea level. (b) Antarctic ice volume. The two vertical dashed lines indicate transitions from 400- to 41-kyr dominant frequencies (~2.9 Myr ago) and from 41- to 100-kyr (~0.9 Myr ago). Power evolution performed with AnalySeries49using a moving window of 1 Myr with intermediate steps of 10 kyr and a Parzen window with 90% lags. Figure 2: Power evolution in eccentricity and obliquity frequency bands. For both panels, 400-kyr power is shown in black, 100-kyr power in red and 41-kyr power in blue. ( a ) Eustatic sea level. ( b ) Antarctic ice volume. The two vertical dashed lines indicate transitions from 400- to 41-kyr dominant frequencies (~2.9 Myr ago) and from 41- to 100-kyr (~0.9 Myr ago). Power evolution performed with AnalySeries [49] using a moving window of 1 Myr with intermediate steps of 10 kyr and a Parzen window with 90% lags. Full size image Coherent variability of ice volume and the carbon cycle Carbon isotope records of both benthic and planktonic foraminiferal δ 13 C data reflect variability in the carbon cycle. For the past glacial cycles they vary out of phase with the benthic δ 18 O data [7] , whereas for long-term pacing δ 13 C and δ 18 O vary in phase [1] , [10] , [11] . Here we have analysed two records over the past 5 Myr, a stacked benthic δ 13 C record from the eastern equatorial Pacific (Leg 138) [13] ( Fig. 1g,h ) and a stacked planktonic δ 13 C record from the Mediterranean [13] . Both sites reflect significant 400-kyr-long eccentricity power ( Supplementary Fig. S3c,f ). In our simulations, the prominent frequency in both AIS volume and eustatic sea level (as calculated from ice-volume change of all four ice sheets) show a clear progression of dominant frequencies in the course of the past 5 Myr ( Fig. 2 ). Notably, prior to inception of the NH ice sheets (~2.9 Myr ago) sea level and AIS variability are dominated by 400-kyr-long eccentricity variability. Around 3–3.5 Myr ago, we observe a short peak in 400-kyr periodicity in the LR04 stack and in the surface-air temperature variations ( Fig. 1b,d ). This has previously been observed and in fact coincides with a node in the 400-kyr power of eccentricity [18] . Following the glacial inception of the NH ice sheets (vertical dashed line in Fig. 2 at 2.9 Myr ago) the sea level progressed into obliquity paced glacial cycles ( Fig. 2a ). The NH ice sheets are predominantly influenced via the SMB that is controlled by local insolation and temperature acting on surface melt [17] . Accordingly, NH ice volume has been shown to be driven by obliquity variations [19] and reflects the dominant obliquity periodicity as shown in the surface temperature ( Fig. 1d and Supplementary Fig. S3b ). The 100-kyr glacial cycles emerge from the NH ice sheets after the Mid-Pleistocene transition (0.9 Myr ago) [20] , [21] . At the same time, the large sea-level fluctuations drive grounding-line advance and retreat of the West AIS. Most remarkable, our simulations show that 400-kyr-long eccentricity cycles are persistently present in the AIS ice volume ( Fig. 2b ) throughout the past 5 Myr. In contrast to the NH ice variations, AIS volume is primarily controlled by sub-shelf processes [17] , [22] . The sub-shelf melt is varied accordingly with surface temperatures and an insolation anomaly ( Supplementary Figs S3,S4 ) to simulate retreat of the West AIS for several interglacial periods [5] , [22] , [23] . The 400-kyr-long eccentricity changes in the δ 13 C data from the Mediterranean and eastern Pacific vary coherently with our simulated AIS throughout the Plio-Pleistocene ( Fig. 3 ). The δ 13 C data lag AIS ice volume with an average of 23.8±0.4 and 54.0±1.6 kyr, respectively ( Fig. 4 ). 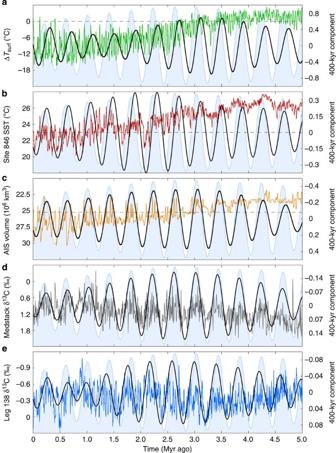Figure 3: Simulated variables and proxies with 400-kyr components. In all panels 400-kyr eccentricity is shown in light-blue shading in the background, 400-kyr filtered component is shown in black (rightyaxis). Horizontal dashed lines represent the PD values. (a) Simulated surface-air temperature anomaly in green. (b) Site 846 Sea Surface Temperature33in red. (c) Simulated Antarctic Ice Sheet ice volume in orange. (d) Mediterranean stack planktonic δ13C data13in grey. (e) Leg 138 benthic δ13C data13in blue. Figure 3: Simulated variables and proxies with 400-kyr components. In all panels 400-kyr eccentricity is shown in light-blue shading in the background, 400-kyr filtered component is shown in black (right y axis). Horizontal dashed lines represent the PD values. ( a ) Simulated surface-air temperature anomaly in green. ( b ) Site 846 Sea Surface Temperature [33] in red. ( c ) Simulated Antarctic Ice Sheet ice volume in orange. ( d ) Mediterranean stack planktonic δ 13 C data [13] in grey. ( e ) Leg 138 benthic δ 13 C data [13] in blue. 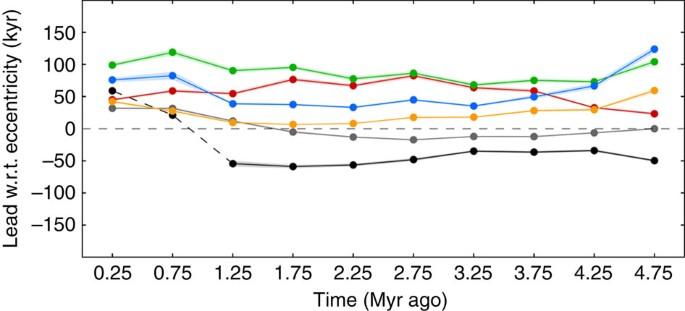Figure 4: Cross-phase analysis of climate variables with eccentricity. Lead (positive) and lag (negative) with respect to the 400-kyr filter of eccentricity. Surface-air temperature in green, Site 846 SSTs33in red, Eustatic sea level in blue, AIS volume in orange, Mediterranean stack planktonic δ13C data13in grey and Leg 138 benthic δ13C data13in black, with the dashed line showing the apparent disappearance of 400-kyr cycles13. Full size image Figure 4: Cross-phase analysis of climate variables with eccentricity. Lead (positive) and lag (negative) with respect to the 400-kyr filter of eccentricity. Surface-air temperature in green, Site 846 SSTs [33] in red, Eustatic sea level in blue, AIS volume in orange, Mediterranean stack planktonic δ 13 C data [13] in grey and Leg 138 benthic δ 13 C data [13] in black, with the dashed line showing the apparent disappearance of 400-kyr cycles [13] . Full size image Sensitivity experiments We have performed eight runs with varying different model parameters as shown in Supplementary Table S1 . All runs have the same basic settings and start 5.32 Myr ago and run to the present day (PD), using the full-time solution of the LR04 benthic δ 18 O stack [16] ( Supplementary Fig. S1 ). First, we have tested the values for the two enhancement factors, constraint by the range as given in Ma et al. [24] Second, the mass balance constant C abl (equation (4)) has been varied for five different sets of values. Uncertainties in ice-flow parameters The use of the shallow ice approximation (SIA) and shallow shelf approximation (SSA) to calculate ice velocities implies an underestimation of ice velocities on land and an overestimation of the velocities in ice shelves [24] . Hence, SIA/SSA ice-sheet-shelf models use enhancement factors to better reproduce ice-flow characteristics, changing ice rheology—that is, the flow parameter for sheet and shelf [24] , [25] . As has been described in Ma et al. [24] , a ratio of E SIA /E SSA between 5 and 10 is considered here. Results show the largest response to changes in the E SSA factor, for which we have tested values between 0.6 and 0.7 ( Supplementary Table S1 ). Responses are largest for the AIS and Greenland ice sheet (GrIS) ( Supplementary Table S2 ), a smaller E SSA factor resulted in a larger AIS during glacial maxima and a smaller GrIS during interglacials—that is, the ice sheets exhibit a greater dynamical response to changes in temperature and/or the sea level. For the Eurasian and North American ice sheets (EuIS and NaIS, respectively), the responses are smaller and are mainly influenced by changing the E SIA factor, which is varied between 4.5 and 5.5. The ranges of these variables correspond to the estimated values given by Ma et al. [24] and are similar to those used in the Parallel Ice Sheet Model (PISM) [25] . Mass balance uncertainties The largest uncertainty in the SMB parameterizations is caused by the calculation of the surface ablation—that is, melt of ice, equation (4). Here we have run the model with five sets of parameters, varying the ablation constant C abl ( Supplementary Table S1 ). In agreement with other studies, a more negative value results in less ablation (reducing the approximate air temperature for which ice starts to melt) [26] . In this case, the NH ice sheets, which are mainly controlled by the SMB, show the largest response of about 5 m sea-level equivalent ( Supplementary Table S2 ), whereas the AIS and GrIS show smaller differences of only a few metres. Overall, these tests show that model results do show a consistent pattern of glacial–interglacial climate variability consistent with the benthic LR04 δ 18 O stack that is used to force the inverse method ( Supplementary Fig. S1 ). In two previous studies with simplified ice-sheet models, but using the same inverse methodology, the uncertainty in model results on other parameterizations were already investigated [27] , [28] . Hence, in Supplementary Fig. S5 the 2σ uncertainty interval is shown, therefore accounting for uncertainties in the benthic δ 18 O data and model parameterizations of deep-ocean temperature and ice-sheet δ 18 O values. Comparison with temperature proxies In Supplementary Fig. S6a–c , we compare our reconstructed surface-air temperature anomaly with three proxy-based sea-surface temperature (SST) estimates from the North Atlantic, Equatorial Pacific and Southern Ocean, respectively. Note that we here compare a surface-air temperature anomaly, derived from a global stacked benthic δ 18 O record, whereas the SST data also include regional variability. The curves are plotted such that the data over the past ~1 Myr largely overlap each other. The overall trends and variability match quite well when compared with these independent proxy-based temperature estimates. All data show a clear overall cooling trend from about 3.5 to 1 Myr ago and strong (100-kyr) glacial–interglacial variability thereafter. Second, we compare our modelled deep-water temperature with an independent reconstruction of deep-water temperature change from the Southern Ocean [29] . The latter is derived from a combination of benthic δ 18 O data and Mg/Ca proxy temperatures. In Supplementary Fig. S7a , we show that the benthic δ 18 O data compare very well with the LR04 benthic stack used in our study. Supplementary Fig. S7b shows the deep-water temperatures, except for the unusually low temperatures around 1.4 Myr ago, our output compares favourably with the proxy-derived estimates. Both data sets show similar values of glacial–interglacial temperature change. Our results indicate that the absence of the 400-kyr-long eccentricity cycles during the Late Pleistocene glacial cycles ( Fig. 1 ) can be ascribed to the dominant variability of the NH ice sheets since 2.9 Myr ago ( Fig. 2a and Supplementary Fig. S3d ), which obscure the 400-kyr variability of the AIS. As has previously been shown, NH ice volume is predominantly controlled through the SMB with the southern margin of the NH ice sheets terminating on land [30] . Henceforth, ice volume is determined by surface melt, induced by insolation and temperature variability [17] . Although NH ice volume also shows 400-kyr variability ( Supplementary Fig. S3d ), this is masked by the much stronger 41- and 100-kyr signals. In contrast, the AIS is mainly influenced by the sea-level change and oceanic melt/refreezing [17] , [22] . Recent studies have shown that sub-shelf melting is also an important contributor to current mass loss of the AIS [31] . The long-term sub-shelf melt variability largely arises from the inclusion of the insolation anomaly (Δ q j ; equation (7)). We have included the insolation anomaly in line with previous studies to simulate retreat of the West AIS [5] , [22] . To test the importance of this hypothesis, we have performed a simulation that does not include the influence of insolation changes on sub-shelf melting ( Supplementary Movie 1 and Supplementary Fig. S4b,c ). The overall climate variability is preserved; however, as is clearly shown the simulated West AIS is not in accordance with observed retreat during several interglacial periods [5] , [23] . Moreover, the 400-kyr power in AIS ice volume is significantly reduced. As a result, the volume is mainly controlled by temperature and sea-level variations ( Supplementary Figs S3,S8 ). Therefore, we can conclude that an insolation-driven process is required to explain the variability of Antarctic ice volume over the Plio-Pleistocene. The connection between AIS variability and the carbon cycle prior to NH glacial inception has been established in the Miocene, for which similar long-term 400-kyr cycles are observed in both oxygen and carbon isotopes [1] , [10] , [11] . During this period, the dominant factor in benthic δ 18 O variability can be ascribed to the AIS [12] , [28] . Analysis of the benthic δ 18 O data has shown that 400-kyr-long eccentricity cycles exist in both simulated AIS volume and temperature [12] . Moreover, Miocene expansion of the AIS has been found to be paced by 400-kyr-long eccentricity cycles, prompting coherent fluctuations in δ 13 C and δ 18 O through the formation of intermediate and deep water [32] . Our simulations reveal that during the past 5 Myr changes in the carbon cycle and in AIS volume vary coherently. Both processes could be driven by low-latitude climate variations, as revealed by the persistent 400-kyr periodicity in both SST from the eastern equatorial Pacific site 846 (ref. 33 ) and the Mediterranean stacked δ 13 C record ( Fig. 3 ) [13] . Our simulated surface-air temperatures (albeit a weakening signal, Fig. 3a ) and the eastern equatorial Pacific SSTs are leading AIS volume and δ 13 C variations ( Fig. 4 ) in support of this hypothesis. This is in agreement with the lag of δ 13 C relative to ice volume as observed before in Miocene isotope data [1] , [11] . Since eccentricity lags rather than leads long-term variability in temperature and AIS volume ( Fig. 4 ), this could imply that the 400-kyr variability emerges from nonlinear processes within the climate system. This nonlinear behaviour is also revealed by the 500-kyr peaks in the benthic δ 13 C data [13] during the past 1 Myr and the disappearance of 400-kyr cycles in the benthic δ 18 O data. For long-term changes, our analysis shows that surface-air temperatures rise in coherence with a reduction in AIS volume and lower δ 13 C. A possible mechanism for this relation is weathering, which could be ascribed to changes in the sea level and the waxing and waning of the AIS [1] . For the past 5 Myr, a coherent relationship has been identified between chemical weathering proxies and benthic δ 13 C data at orbital time scales, indicating that an increase in chemical weathering may result in lower δ 13 C and a pCO2 increase [34] . During the Pleistocene, however, sea-level changes are largely controlled by NH ice volume. Hence, the NH ice sheets presumably played a significant role on variability in weathering. Likewise, the marked increase in AIS volume at the Eocene–Oligocene transition has been linked to a drawdown in δ 13 C and weathering conditions as well [35] . In conclusion, our simulations of ice volume over the past 5 Myr support previous theories that have been put forward on the overriding influence of the NH ice sheets after the Mid-Pleistocene transition on the δ 13 C spectral properties. We have shown for the first time that the long-term changes of Antarctica reveal the persistent interaction between ice sheets, the ocean and the carbon cycle. Notwithstanding, we present a qualitative interpretation and a more comprehensive case could be made when using a coupled system that includes both climate and carbon-cycle models. Our results do show that Antarctic ice volume and carbon-cycle dynamics vary coherently, which can now be traced back into the Miocene and allows for a new understanding of the ‘400-kyr problem’. Calculating ice volume and temperature from benthic δ 18 O data Benthic δ 18 O data are a proxy for global ice volume and deep-water temperature [15] . We use an inverse forward modelling approach to deduce ice volume and temperature from the LR04 benthic δ 18 O record [16] . Here we assume that deep-water temperatures and ice volume are related to changes in the surface-air temperature over the NH. The NH temperature anomaly drives the changes in ice volume over Eurasia and North America and controls deep-water formation [36] . The approach derives the NH temperature anomaly from the difference between the modelled and observed benthic δ 18 O data [17] . The ice-volume contribution follows from mass conservation of δ 18 O between the ocean and ice sheets [17] . Deep-water temperature anomalies are linearly related to the surface-air temperature anomaly [36] and the contribution to benthic δ 18 O data follows from a palaeotemperature parameterization [37] . From this approach, we derive a continuous and self-consistent record of surface-air temperature, ice volume and benthic δ 18 O data ( Supplementary Fig. S1a–c ). This methodology has been applied in several studies that investigate ice-volume evolution during the late Cenozoic [17] , [20] , [28] , [36] . A full description of the approach can be read in de Boer et al. [17] Simulating global ice volume The NH temperature anomaly is forwarded to four 3D ice-sheet-shelf models and applied to the SMB fields. To allow for long million-year simulations, ice velocities are computed using approximate solutions of the stress balance for sheet and shelf flow, including a representation of the transition zone from sheet to shelf [17] . Surface and basal mass balance are accounted for by parameterizations that include changes in temperature and solar insolation. Subsequently, the total mass budget of the ice sheet is closed with ice discharge towards open water. Ice fluxes and mass continuity The ANICE ice-sheet-shelf model is based on the SIA for sheet flow on land [38] and the SSA for ice streams and shelves [39] . Following the approach that has been put forward in the PISM [40] , the SSA velocities are used to determine sliding velocities and are added to the SIA velocities such that a smooth transition is obtained for ice-flow from sheet to shelf [41] . Both velocities are adjusted with an enhancement factor E SIA and E SSA , for which the default values are chosen to be 5.0 and 0.7, respectively, close to the values as used in PISM [25] , and within the range as determined in a recent study [24] . The mass continuity equation is given by: with H i being the ice thickness (in m), Q the ice flux (m 2 per year) and B the mass balance (m per year), given by the SMB and sub-shelf melt or refreezing. The ice flux Q is divided in a diffusive (SIA) and SSA part as: With the diffusivity D being the scalar part from the SIA velocity equation [17] , and H s the surface elevation (in m). Velocities are calculated on the regular ice thickness grid points, from which the ice fluxes are determined in between grid points A and B (staggered) using a centred difference discretization: In the SSA term, ice thickness Hi is chosen to be Hi A if the average SSA velocity between point A and B is positive, if negative, Hi is chosen to be Hi B . The rectangular grid size is 20 km for the GrIS and 40 km for the EuIS, NaIS and AIS. For each grid point, the fluxes towards the directly adjacent grid points are calculated as outgoing fluxes. To keep mass conserved, in case the mass balance is negative and larger than the available ice thickness at the grid point, the outgoing fluxes are set to zero and the mass balance is set equal to the available ice thickness. After the mass conservation check, the outgoing fluxes are reduced if the combined flux exceeds the sum of the available ice thickness and mass balance (either negative or positive) during that specific time step. The total mass balance of the ice sheet is conserved and per definition is calculated from the SMB (positive or negative), the sub-shelf mass balance (positive or negative) and ice discharge towards open ocean points (negative). Mass conservation over the entire domain is monitored and is negligible during the entire 5.32 Myr simulation. The SMB For the SMB, the initial precipitation and temperature fields are taken from the ERA-40 Reanalysis data set [42] , using monthly averaged fields from 1971 to 2000. Accumulation over Greenland and Antarctica is adjusted according to changes in temperature, following the Clausius–Clapeyron relation [17] . A precipitation model has been used for the two large NH ice sheets to adjust the PD precipitation fields. The model includes orographic forcing of precipitation and changes in the moisture content, which are calculated from the 2-m surface-air temperature and the 850-hPa wind fields [17] . The melt rate (in m w.e. per year) is calculated from a parameterization that is based on PD mass balance observations and modelling results for Antarctica and Greenland and incorporates changes in temperature and insolation: here Q is the monthly incoming shortwave radiation at the top of the atmosphere (W m −2 ), which is changed every 1,000 years [43] , 0.513 is an average value for the transmissivity of the atmosphere and α is the albedo of the surface. Furthermore, ρ fw is the density of fresh water, L is the latent heat of fusion (both shown in Supplementary Table S3 ) and Δ t is the time step of the melt model—that is, a month. The constant 10 (W m −2 K −1 ) shows the dependence on the temperature, and C abl is a constant that is set to −32 W m −2 for the AIS and the two NH ice sheets. For Greenland, this value is set to −40 W m −2 . These values are chosen in such a way that after several glacial cycles the PD ice volume closely matches the current observations of ice volume, and the PD SMB patterns are in agreement with observations. The parameterization can only produce positive values—that is, melt of ice—and also accounts for the importance of changes in the solar insolation when calculating ablation [44] . Sub-shelf melt or refreezing The calculation of sub-shelf melt or refreezing in ANICE uses a combination of several parameterizations introducing glacial–interglacial changes and ice shelves that show close to PD extent [22] , [25] . For the GrIS model, ice shelves are considered negligible and are not taken into account. Underneath the ice shelves, the melt rate is based on heat transfer between the bottom of the ice and the ocean water [25] , [45] : with the different parameters adopted from PISM [25] and shown in Supplementary Table S3 . Here ρ w is the seawater density (kg m −3 ), c pO is the specific heat capacity of the ocean (J kg −1 °C −1 ), γ T is the thermal exchange velocity (m s −1 ), F melt the sub ice-shelf melt parameter (m s −1 ), L the Latent heat of fusion (J kg −1 ) and ρ i the density of ice. T oc is the ocean-water temperature (°C) adjusted with a weighting function (equation (7)). The melt rate can have both positive and negative values, either leading to melting of ice shelves or (re)freezing of ocean water [45] . The freezing temperature of the saline ocean water (in °C) at the shelf base is calculated with: with S O =35 psu being the average salinity of the ocean water and z b being the depth of the ice-shelf base (in m) calculated as: z b =−(ρ i /ρ w )H i. To simulate glacial–interglacial climate variability, the ocean temperature T oc in equation (5) is adjusted with a weighting function, including changes in temperature and a small influence of summer insolation [22] : Here Δ T is the applied temperature anomaly relative to PD. Furthermore, Δ q j is the summer insolation anomaly relative to PD, using the January 80 °S anomaly for the AIS, and the June 65°N anomaly (W m −2 ) for the large NH ice sheets. The ocean temperature is then adjusted for colder than PD periods, when 0≤ w g <1, as: and for warm periods, when 1≤ w g ≤2: T CD , T PD and T WM indicate the cold, PD and warm values of the uniform ocean temperature as shown in Supplementary Table S3 . These values are applied to the ice sheets as spatial uniform values and are based on values found in climate models and observations [46] , [47] . How to cite this article: de Boer, B. et al. Persistent 400,000-year variability of Antarctic ice volume and the carbon cycle is revealed throughout the Plio-Pleistocene. Nat. Commun. 5:2999 doi: 10.1038/ncomms3999 (2014).